Gap junction signalling is a stress-regulated component of adrenal neuroendocrine stimulus-secretion couplingin vivo Elucidating the mechanisms whereby neuroendocrine tissues coordinate their input and output signals to ensure appropriate hormone secretion is currently a topical issue. In particular, whether a direct communication mediated by gap junctions between neurosecretory cells contributes to hormone release in vivo still remains unknown. Here we address this issue using a microsurgical approach allowing combined monitoring of adrenal catecholamine secretion and splanchnic nerve stimulation in anaesthetised mice. Pharmacological blockade of adrenal gap junctions by the uncoupling agent carbenoxolone reduces nerve stimulation-evoked catecholamine release in control mice and to a larger extent in stressed mice. In parallel, the gap junction-coupled cell network is extended in stressed mice. Altogether, this argues for a significant contribution of adrenomedullary gap junctions to catecholamine secretion in vivo . As such, gap junctional signalling appears to be a substantial component for neuroendocrine function in the adrenal medulla, as it may represent an additional lever regulating hormone release. Hormone secretion from neuroendocrine tissues is a highly regulated process that needs a finely tuned coordination between incoming and output signals. In this regard, adrenal chromaffin cells are remarkable and the study of their secretory machinery [1] , [2] and more recently of their synaptic inputs [3] , [4] , [5] has contributed substantially to the current knowledge on cellular mechanisms underlying neurosecretion function. However, compelling evidence obtained in acute adrenal slices indicates that neurosecretory mechanisms are more intricate than previously envisioned. Indeed, catecholamine release appears to be dualistically controlled by an incoming initial command assisted by local modulation [6] , [7] , supporting the hypothesis of an amplifying system occurring at the chromaffin cell level [8] . The command triggering catecholamine secretion comes from the sympathetic nervous system synapsing onto chromaffin cells. Under basal condition (low splanchnic nerve frequency discharge), acetylcholine (ACh) is the primary neurotransmitter released at the splanchnic nerve terminal-chromaffin synapse. In response to stress or emergency conditions associated with a high nerve frequency firing, a dual splanchnic-adrenal neurotransmission involving both ACh and the pituitary adenylate cyclase-activating polypeptide PACAP occurs [9] , [10] , thus enhancing chromaffin cell secretion. In complement to synaptic transmission, direct communication through gap junctions between chromaffin cells ensures propagation of electrical and ensuing calcium signals between neurosecretory cells and amplifies catecholamine release in response to stimulation of a single cell [11] . The differential regulation of gap junctions and cholinergic synapses cells in physiolological and pathological conditions associated with specific catecholamine demand, such as during early postnatal development [4] , [12] and in response to chronic stress [13] , [14] , is indicative of a functional interaction between incoming commands and local communication and points towards a putative contribution of gap junctions to stimulus-secretion coupling. Converging arguments have been accumulated that strongly support this hypothesis, but the ex vivo acute slice preparation used to obtain them does not allow a definitive demonstration. We present here a new experimental approach to simultaneously monitor the electrical activity of chromaffin cells and catecholamine secretion in response to splanchnic nerve stimulations in anaesthetised adult mice. This in vivo technique is combined with a series of histological and molecular analysis of gap junction protein connexins and of dye diffusion through gap junctions in control, cold-stressed and connexin-deficient animals. We demonstrate that adrenal gap junctional signalling contributes positively to catecholamine release in response to splanchnic nerve stimulation in vivo . Furthermore, this contribution is enhanced in stressed animals, providing an additional level of regulation for stimulation-secretion coupling in the adrenal gland. Electrical activity in the mouse adrenal gland in vivo To determine the contribution of gap junctions to stimulus-secretion coupling in anaesthetised mice, blood from the left adrenal gland was collected during electrical stimulation of the splanchnic nerve ( Fig. 1a and Supplementary Fig. S1 ; Supplementary Movie 1 ). The electrical behaviour of the adrenal medullary tissue was monitored using a microelectrode implanted into the adrenal medulla (location identified by injection of Chicago Sky Blue 6B; Supplementary Fig. S2 ). A spontaneous electrical activity was observed ( Fig. 1b , recording duration: 9–22 min, mean frequency 0.87±0.26 Hz (mean±s.e.m., n =9 mice)). It consisted of a continuous firing on which intermittent bursts were superposed in 7/9 mice (1–8 min duration, intra-burst frequency 2.7±1.1 Hz (mean±s.e.m.)). Tetrodotoxin (TTX, 3 μM) applied locally on the splanchnic nerve induced a marked (89±3.5% (mean±s.e.m., n =9 mice)) and partially reversible decrease of the firing activity ( Fig. 1c ), indicating that the in vivo spontaneous firing of the mouse adrenal medulla mainly results from excitatory afferent inputs. 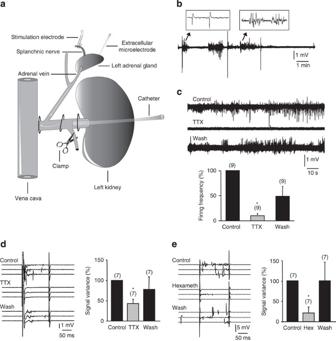Figure 1:In vivorecording of spontaneous and splanchnic nerve stimulation-evoked electrical activity. (a) Experimental protocol used to simultaneously monitor intra-adrenal electrical activity and collect blood outflow from the adrenal vein. (b) Spontaneous electrical activity recorded in the medullary tissue comprising both individual spikes (left inset) and bursting activities (right inset). (c) Reversible blockade of spontaneous activity by 3 μM TTX locally applied on the nerve. *P<0.05 versus control, Mann–WhitneyU-test,n=9 mice. Values represent mean±s.e.m. (d,e). Reversible decrease of splanchnic nerve stimulation-evoked electrical activity (10 V, 160 ms, 3 iterations, 1/min), in response to TTX (d,n=7 mice) and to hexamethonium (e, 200 μM, injection through the recording pipette,n=7 mice). *P<0.05 versus control, Mann–WhitneyU-test. Values represent mean±s.e.m. Figure 1: In vivo recording of spontaneous and splanchnic nerve stimulation-evoked electrical activity. ( a ) Experimental protocol used to simultaneously monitor intra-adrenal electrical activity and collect blood outflow from the adrenal vein. ( b ) Spontaneous electrical activity recorded in the medullary tissue comprising both individual spikes (left inset) and bursting activities (right inset). ( c ) Reversible blockade of spontaneous activity by 3 μM TTX locally applied on the nerve. * P <0.05 versus control, Mann–Whitney U- test, n =9 mice. Values represent mean±s.e.m. ( d , e ). Reversible decrease of splanchnic nerve stimulation-evoked electrical activity (10 V, 160 ms, 3 iterations, 1/min), in response to TTX ( d , n =7 mice) and to hexamethonium ( e , 200 μM, injection through the recording pipette, n =7 mice). * P <0.05 versus control, Mann–Whitney U- test. Values represent mean±s.e.m. Full size image Splanchnic nerve stimulation (10 V, 160 ms) triggered a burst of bipolar action potentials occurring specifically during the stimulation ( Fig. 1d , upper traces). In the seven mice recorded, application of 3 μM TTX onto the nerve significantly decreased the evoked activity ( Fig. 1d , middle traces), as illustrated by the decreased variance of the signal. This unambiguously shows that evoked electrical activity in the medullary tissue results from action potentials running along the splanchnic nerve and not from a direct activation of the gland. In addition, this activity was reversibly inhibited (by 78±12% (mean±s.e.m., n =7 mice)), by a local injection of hexamethonium, an antagonist of α3-built nAChRs, through the recording pipette (200 μM, Fig. 1e ). This demonstrates the involvement of cholinergic synaptic terminals, as expected for splanchnic nerve-evoked activity, and the dominant contribution of nAChRs rather than muscarinic receptors. Basal and nerve stimulation-evoked catecholamine release To go further in characterizing excitation-secretion coupling in the adrenal medulla in vivo , we measured catecholamine secretion, at rest and in response to splanchnic nerve stimulation ( Fig. 1a for a schematic illustration of the protocol, Supplementary Fig. S1 and Supplementary Movie 1 for direct visualization). Basal plasma norepinephrine (NE) and epinephrine (E) were assayed in blood samples collected from the left adrenal vein during 2 or 5 min. No statistical difference was observed between catecholamine concentrations measured using the two sampling durations (NE: 15.4±2.9 nM (mean±s.e.m., n =11 mice) for 2 min and 25.1±5.2 nM (mean±s.e.m., n =17 mice) for 5 min, P >0.05, Mann–Whitney U -test; E: 318±111 nM (mean±s.e.m., n =11 mice) for 2 min and 384±177 nM (mean±s.e.m., n =17 mice) for 5 min, P >0.05, Mann–Whitney U -test). We next examined splanchnic nerve stimulation-evoked catecholamine secretion. Two protocols were used: a low frequency (LF, 0.1 Hz, 5 min) to mimic basal tone firing and a high frequency (HF, 4 Hz, 2 min) to mimic stress firing conditions [15] . Two blood samples were successively collected, a control (C) one first and then a test (T)one during nerve stimulation. In the absence of stimulation, NE and E concentrations in the two successive samples did not significantly differ (NE: C=36.6±8.5 nM (mean±s.e.m.) and T=55.7±22.7 nM (mean±s.e.m., n =12 mice), P >0.05, Mann–Whitney U -test; E: C=459±241 nM (mean±s.e.m.) and T=500±297 nM (mean±s.e.m., n =12 mice), P >0.05, Mann–Whitney U -test). Both LF and HF splanchnic nerve stimulations triggered a frequency-dependent release of catecholamines (>twofold and >10-fold for NE and E, respectively, Fig. 2 ). It is noteworthy that not only basal but also evoked E release is much larger than NE release. This is consistent with the fact that mouse chromaffin cells mainly exhibit an adrenergic phenotype (80% of epinephrine-containing cells [16] ). 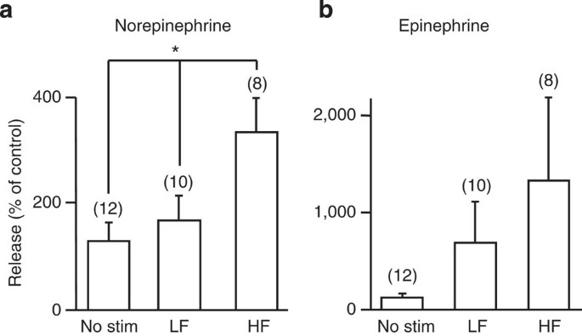Figure 2: Stimulus frequency-dependent catecholamine secretion. Ratio between catecholamine concentrations before (C) and after (T) splanchnic nerve stimulation. In the absence of stimulation (no stim), T/C was slightly but not significantly higher than 100%. LF and HF columns indicate increased NE (a) and E (b) concentrations in response to graded stimulation. LF, low frequency (0.1 Hz, 160 ms, 10 V, 5 min), HF, high frequency (4 Hz, 1 ms, 10 V, 2 min). *P<0.05, two-way analysis of variance (followed by Bonferroni’spost hoctest). Values represent mean±s.e.m. The number of recorded mice for each condition is indicated in parentheses. Figure 2: Stimulus frequency-dependent catecholamine secretion. Ratio between catecholamine concentrations before (C) and after (T) splanchnic nerve stimulation. In the absence of stimulation (no stim), T/C was slightly but not significantly higher than 100%. LF and HF columns indicate increased NE ( a ) and E ( b ) concentrations in response to graded stimulation. LF, low frequency (0.1 Hz, 160 ms, 10 V, 5 min), HF, high frequency (4 Hz, 1 ms, 10 V, 2 min). * P <0.05, two-way analysis of variance (followed by Bonferroni’s post hoc test). Values represent mean±s.e.m. The number of recorded mice for each condition is indicated in parentheses. Full size image Contribution of gap junctions to catecholamine release The mouse adrenal medullary tissue was much more immunoreactive to Cx36 than to Cx43 ( Fig. 3a ). The opposite situation was observed in the cortex. Gap junction involvement in nerve stimulation-evoked catecholamine release was determined by blocking junctional coupling. Mice were injected i.p . at the beginning of the surgical procedure with either NaCl (9‰), the uncoupling agent carbenoxolone (CBX, 100 mg kg −1 ) or its inactive structural analogue glycyrrhizic acid (GZA, 135 mg kg −1 ). CBX injection significantly reduced gap junctional coupling in the adrenal gland, as evidenced by decreased diffusion of the fluorescent dye Lucifer yellow (LY) measured by scrape loading [13] ( Fig. 3b ). In mice injected with GZA ( n =11) or NaCl ( n =8), LY widely diffused from the cut edge of the gland into the cortex and medulla, whereas, in mice injected with CBX ( n =5), diffusion was greatly decreased and LY accumulated on the cut edge of the medulla ( Fig. 3b ). Quantification of LY diffusion into the gland ( Fig. 3c and d ) indicates a reduced (25.8% decrease) diffusion in the depth of the gland in CBX-treated mice. Similarly, CBX treatment (5 mice) reduced by 30.5% Alexa Fluor 594-conjugated cadaverine diffusion when compared with GZA ( n =7 mice, P <0.05, Mann–Whitney U -test, Fig. 3d and Supplementary Fig. S3 ). These findings unambiguously show the presence of functional gap junctions in the mouse adrenal medullary tissue and demonstrate the efficiency of CBX to block gap junctional coupling in our experimental conditions. 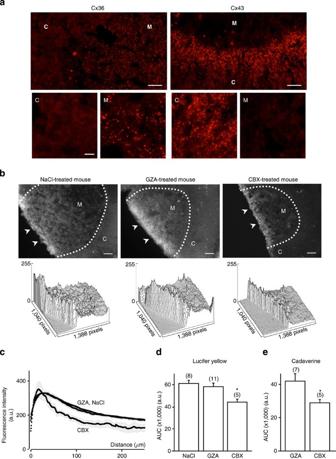Figure 3: Significant reduction of fluorescent dye diffusion in the adrenal gland afteri.p.injection of carbenoxolone. (a) Cx36 and Cx43 immunostainings showing that Cx36 is specifically expressed in the medulla, whereas the cortex displays a robust labelling for Cx43. Scale bar, 50 μm. The punctuate fluorescent staining typical of a gap junction marker is evidenced at higher magnification (scale bar, 10 μm). (b–d) Intra-peritoneal injection of carbenoxolone (CBX, 100 mg kg−1) attenuates LY diffusion when compared with glycyrrhyzic acid (GZA, 135 mg kg−1) or NaCl (9‰). (b) Representative snapshots (scale bar, 100 μm) and associated wireframe plots illustrating the cutting edge. Quantification of LY diffusion measured as the fluorescence intensity versus distance from the edge (c) and as the area under this curve (d, *P<0.05 versus GZA, Mann–WhitneyU-test,n=5 CBX- and 11 GZA-injected animals. Values represent mean±s.e.m.). (e). Quantification measured as the area under the curve of Alexa Fluor 594-conjugated Cadaverine diffusion in GZA- and CBX-injected mice showing that CBX significantly reduced cadaverine diffusion extent within the adrenal gland. *P<0.05 versus GZA, Mann–WhitneyU-test,n=5 CBX- and 7 GZA-injected mice. Values represent mean±s.e.m. Figure 3: Significant reduction of fluorescent dye diffusion in the adrenal gland after i.p. injection of carbenoxolone. ( a ) Cx36 and Cx43 immunostainings showing that Cx36 is specifically expressed in the medulla, whereas the cortex displays a robust labelling for Cx43. Scale bar, 50 μm. The punctuate fluorescent staining typical of a gap junction marker is evidenced at higher magnification (scale bar, 10 μm). ( b – d ) Intra-peritoneal injection of carbenoxolone (CBX, 100 mg kg −1 ) attenuates LY diffusion when compared with glycyrrhyzic acid (GZA, 135 mg kg −1 ) or NaCl (9‰). ( b ) Representative snapshots (scale bar, 100 μm) and associated wireframe plots illustrating the cutting edge. Quantification of LY diffusion measured as the fluorescence intensity versus distance from the edge ( c ) and as the area under this curve ( d , * P <0.05 versus GZA, Mann–Whitney U- test, n =5 CBX- and 11 GZA-injected animals. Values represent mean±s.e.m.). ( e ). Quantification measured as the area under the curve of Alexa Fluor 594-conjugated Cadaverine diffusion in GZA- and CBX-injected mice showing that CBX significantly reduced cadaverine diffusion extent within the adrenal gland. * P <0.05 versus GZA, Mann–Whitney U- test, n =5 CBX- and 7 GZA-injected mice. Values represent mean±s.e.m. Full size image Further, we performed similar scrape-loading experiments using mefloquine (MFQ), another gap junction uncoupling agent potently active on Cx36-built gap junction channels [17] . When compared with vehicle (10 glands from 5 mice), MFQ (25 mg kg −1 ) significantly reduced (by 22.7%) LY diffusion throughout the adrenal gland ( n =14 glands from 7 mice, P <0.05, Mann–Whitney U -test, Supplementary Fig. S4A-C ). It is of note that this percentage is comparable to that obtained in CBX-treated mice ( Fig. 3d ). Is catecholamine secretion (at rest and in response to splanchnic nerve stimulation) altered when gap junctional communication is reduced? First, basal catecholamine release is significantly higher in mice treated with GZA, CBX, MFQ or its vehicle than in NaCl-injected mice ( Supplementary Fig. S5 ). However, MFQ by itself did not significantly enhance basal catecholamine concentration when compared with its vehicle. Because GZA and CBX have been previously described as hypertensinogenic compounds when infused intra-cerebroventricularly [18] , we investigated whether GZA, CBX and MFQ were able to modify arterial blood pressure under our experimental conditions. Systolic arterial blood pressure (SBP) was measured by tail-cuff plethysmography in anaesthetised mice either not injected (sham) or injected with NaCl, GZA, CBX, vehicle or MFQ. As illustrated in Supplementary Fig. S6 , neither CBX nor GZA increased SBP in our conditions. Conversely, when compared with control values measured before drug injection, CBX, GZA and MFQ decreased SBP by significant values (Mann–Whitney U -test) for CBX (24.6%) and MFQ (27.4%). This suggests that the increased basal catecholamine secretion measured in the adrenal-venous blood in response to GZA, CBX and MFQ might be a functionally adaptive response to counteract a hypotension-induced stress. It is also of note that none of the injected compounds altered cardiac frequency during the recording period. The contribution of gap junctions to splanchnic nerve stimulation-evoked catecholamine release was addressed by comparing the T/C ratio in CBX- and GZA-injected mice. Indeed, as GZA and CBX affected basal release to the same extent, the action of CBX on nerve stimulation-evoked release was measured by comparison with that of GZA. As illustrated in Fig. 4 , CBX decreased both NE and E release evoked by a LF ( Fig. 4a ) or HF ( Fig. 4b ) stimulation, although a statistically significant difference was found only for NE release triggered by HF stimulation (58% decrease, n =9 GZA- and 8 CBX-treated mice, P <0.05, Mann–Whitney U -test). Similarly, MFQ trended to decrease HF stimulation-evoked NE release (47% decrease, n =5 vehicle- and 9 MFQ-injected mice, P >0.05, Mann–Whitney U -test) without affecting epinephrine release ( Supplementary Fig. S4D ). This finding demonstrates that gap junction-mediated intercellular communication in the adrenal gland has a notable contribution to hormone release, at least NE, in vivo . 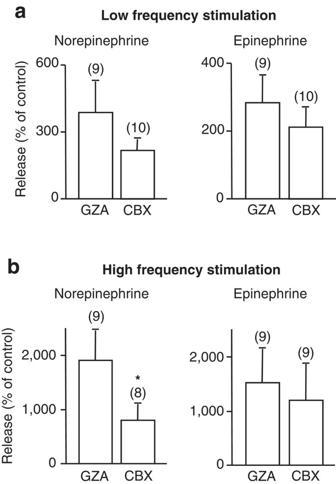Figure 4: Effect of carbenoxolone on stimulation-evoked catecholamine secretion. (a) CBX modifies neither NE nor E release triggered by LF stimulation (n=9–10 mice. Values represent mean±s.e.m.). (b) Significant CBX-induced decrease in NE secretion evoked by HF stimulation (*P<0.05 versus GZA, Mann–WhitneyU-test,n=8–9 mice. Values represent mean±s.e.m.). Figure 4: Effect of carbenoxolone on stimulation-evoked catecholamine secretion. ( a ) CBX modifies neither NE nor E release triggered by LF stimulation ( n =9–10 mice. Values represent mean±s.e.m.). ( b ) Significant CBX-induced decrease in NE secretion evoked by HF stimulation (* P <0.05 versus GZA, Mann–Whitney U- test, n =8–9 mice. Values represent mean±s.e.m.). Full size image Increased contribution of gap junctions in stressed mice We next investigated the effect of CBX in a condition in which gap junctions are increased. The procedure was identical as in our previous work [13] , [14] , in which we have demonstrated that a chronic systemic stress (cold exposure) induces a persistent increase in gap junctional coupling between chromaffin cells and upregulates both Cx36 and Cx43 expression in rat. As the effects of chronic stress may last several hours or days after the end of the stressful stimulus, they can be studied in an animal killed or anaesthetized immediately after return to normal conditions. As illustrated in Fig. 5a , Cx36 immunostaining in the adrenal medulla was twofold higher in cold-stressed ( n =6 mice) than in control ( n =5) mice ( P <0.05, Mann–Whitney U -test). It is noteworthy that expression of Cx43, dominant in the cortex, was not changed by stress ( Supplementary Fig. S7 ). LY diffusion was significantly reduced in CBX- as compared with GZA-injected mice ( Fig. 5b and associated wireframe plots). This reduction (51.2%, Fig. 5c and d ) is greater than that in control mice ( Fig. 3d ). Altogether, these data are consistent with a robust increase of medullary gap junction-mediated cell-to-cell communication in cold-stressed mice. Basal plasma NE and E concentrations were surprisingly lower in cold-stressed mice than in unstressed mice ( Supplementary Fig. S5 ). However, as these basal concentrations remained similar for CBX- and GZA treatments, contribution of gap junctions to stimulus-secretion coupling could be evaluated by comparing nerve-evoked release after these two treatments. As illustrated in Fig. 6 , CBX decreased HF stimulation-evoked NE release to a larger extent in cold-stressed than in control mice (reduction by 76% in stressed mice, n =11 animals, as compared with 58% in control mice ( n =11), P <0.05, Mann–Whitney U -test). In addition, while CBX did not significantly affect E release in control mice (21% reduction), it reduced markedly E secretion in cold-stressed mice (75% reduction, n =11 GZA- and 11 CBX-injected animals, P <0.05, Mann–Whitney U -test). Altogether, data obtained in control and cold-stressed mice demonstrate the contribution of adrenal medullary gap junctions to splanchnic nerve stimulation-evoked catecholamine secretion in vivo , and their predominant involvement in stressful situations. 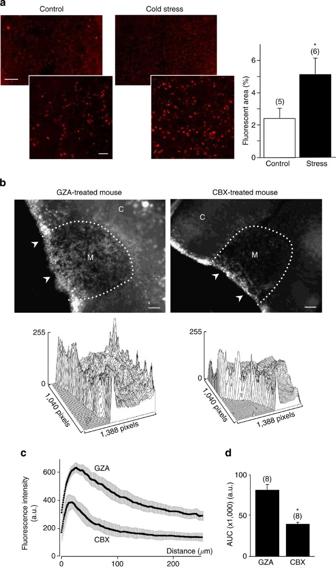Figure 5: Carbenoxolone-induced reduction of Lucifer yellow diffusion in the adrenal gland of cold-stressed mice. (a). Significant increase of Cx36 immunolabelling in the medulla. Scale bar, 50 μm. Inset is at higher magnification (scale bar, 10 μm). *P<0.05 versus control, Mann–WhitneyU-test,n=5 control mice and 6 cold-stressed mice. Values represent mean±s.e.m. (b–d). Scrape-loading data illustrating the CBX-induced reduction of LY diffusion. (b) Representative snapshots (scale bar, 100 μm) and wireframe plots. (c) Quantification of LY diffusion measured as the fluorescence intensity versus distance from the edge. (d) Quantification of LY diffusion measured as the area under this curve (d, *P<0.05 versus GZA, Mann–WhitneyU-test,n=8 GZA- and 8 CBX-treated mice. Values represent mean±s.e.m.). Figure 5: Carbenoxolone-induced reduction of Lucifer yellow diffusion in the adrenal gland of cold-stressed mice. ( a ). Significant increase of Cx36 immunolabelling in the medulla. Scale bar, 50 μm. Inset is at higher magnification (scale bar, 10 μm). * P <0.05 versus control, Mann–Whitney U- test, n =5 control mice and 6 cold-stressed mice. Values represent mean±s.e.m. ( b – d ). Scrape-loading data illustrating the CBX-induced reduction of LY diffusion. ( b ) Representative snapshots (scale bar, 100 μm) and wireframe plots. ( c ) Quantification of LY diffusion measured as the fluorescence intensity versus distance from the edge. ( d ) Quantification of LY diffusion measured as the area under this curve ( d , * P <0.05 versus GZA, Mann–Whitney U- test, n =8 GZA- and 8 CBX-treated mice. Values represent mean±s.e.m.). 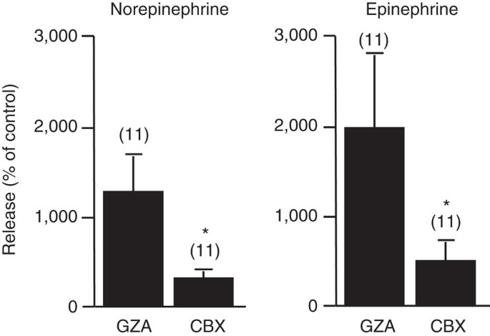Figure 6: Effect of carbenoxolone on stimulation-evoked catecholamine secretion in cold-stressed mice. Intra-peritoneal CBX injection (n=11 animals) induced a robust decrease in both NE and E secretion evoked by a HF stimulation (*P<0.05 versus GZA (n=11 animals), Mann–WhitneyU-test. Values represent mean±s.e.m.). Full size image Figure 6: Effect of carbenoxolone on stimulation-evoked catecholamine secretion in cold-stressed mice. Intra-peritoneal CBX injection ( n =11 animals) induced a robust decrease in both NE and E secretion evoked by a HF stimulation (* P <0.05 versus GZA ( n =11 animals), Mann–Whitney U- test. Values represent mean±s.e.m.). Full size image Impaired nerve stimulation-evoked secretion in Cx36 −/− mice Stimulus-secretion coupling was also investigated in Cx36-deficient (Cx36 −/− ) mice. As expected, the transcript encoding Cx36 was robustly expressed in wild-type mice but not detected in Cx36 −/− mice, whereas Cx43 mRNA expression was similar in wild-type and Cx36 −/− mice ( Fig. 7a ). Interestingly, the expression of mRNA encoding Cx29, a connexin expressed in S100-positive medullary cells [6] , was significantly enhanced in Cx36 −/− mice. Expression of Cx36 and Cx43 proteins was also assessed by immunohistofluorescence ( Fig. 7b ). In glands from Cx36 −/− mice, Cx36 was detected neither in the cortex nor in the medulla. Cx43 was not detected in the medulla but was expressed in the cortex, at a level comparable to that in control mice (6.7±0.5 AU (mean±s.e.m., n =11 glands from 6 mice) for Cx36 −/− and 7.5±1.1 AU (mean±s.e.m., n =11 glands from 6 mice) for wild type, P >0.05, unpaired Student’s t -test). 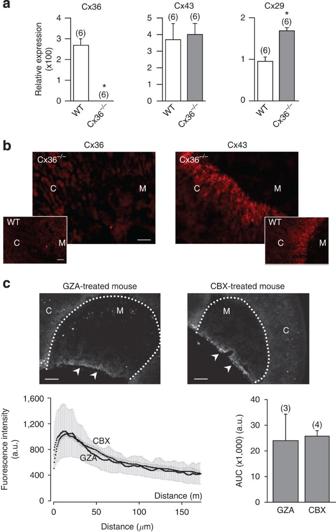Figure 7: Carbenoxolone fails to reduce Lucifer yellow diffusion in the adrenal medulla of Cx36−/−mice. (a) Quantitative RT-PCR illustrating connexin expression in wild-type (WT,n=6 mice) and Cx36−/−mice (n=6) macrodissected medulla. Data confirm invalidation of theCx36gene. While expression of Cx43 transcripts is not modified in Cx36−/−mice, Cx29 transcript is upregulated (*P<0.05 versus WT, Mann–WhitneyU-test. Values represent mean±s.e.m.). (b) Immunohistofluorescence images obtained from Cx36−/−(large photographs, scale bar, 50 μm) and WT (insets, scale bar, 10 μm) mice show that Cx36 is absent from the medulla of Cx36−/−mice, and that Cx43 is exclusively detected in the cortex of Cx36−/−and WT animals. (c) Scrape-loading data (scale bar, 100 μm) and associated analyses show that CBX failed to reduce LY diffusion in adrenal glands of Cx36−/−mice (Mann–WhitneyU-test,n=3 GZA- and 4 CBX-treated mice. Values represent mean±s.e.m.). Figure 7: Carbenoxolone fails to reduce Lucifer yellow diffusion in the adrenal medulla of Cx36 −/− mice. ( a ) Quantitative RT-PCR illustrating connexin expression in wild-type (WT, n =6 mice) and Cx36 −/− mice ( n =6) macrodissected medulla. Data confirm invalidation of the Cx36 gene. While expression of Cx43 transcripts is not modified in Cx36 −/− mice, Cx29 transcript is upregulated (* P <0.05 versus WT, Mann–Whitney U- test. Values represent mean±s.e.m.). ( b ) Immunohistofluorescence images obtained from Cx36 −/− (large photographs, scale bar, 50 μm) and WT (insets, scale bar, 10 μm) mice show that Cx36 is absent from the medulla of Cx36 −/− mice, and that Cx43 is exclusively detected in the cortex of Cx36 −/− and WT animals. ( c ) Scrape-loading data (scale bar, 100 μm) and associated analyses show that CBX failed to reduce LY diffusion in adrenal glands of Cx36 −/− mice (Mann–Whitney U- test, n =3 GZA- and 4 CBX-treated mice. Values represent mean±s.e.m.). Full size image Scrape-loading experiments show an accumulation of LY at the cut edge of the gland and equal diffusion of the dye within the gland of GZA- and CBX-treated Cx36 −/− mice ( Fig. 7c , n =3 GZA- and 4 CBX-injected mice). These data are consistent with a lack of LY-permeable gap junctions in the medulla of Cx36 −/− mice and strengthen a dominant expression of Cx36 in the mouse adrenal medulla. Basal catecholamine release was comparable between CBX- and GZA-treated Cx36 −/− mice and similar to the basal release in control mice ( Supplementary Fig. S5 ). However, counter to expectations, HF nerve stimulation did not evoke any significant catecholamine release in Cx36 −/− mice, whatever the treatment with GZA or CBX ( Fig. 8 ). To try and understand the failure of nerve stimulation to evoke catecholamine release, we tested for integrity of nerve endings and synapses. Nerve terminals were visualized with antibodies against heavy neurofilaments (NF, 200 kDa) to label nerve fibres and against the vesicular acetylcholine transporter (VAChT) to detect synaptic vesicles. As illustrated in Fig. 9a , both NF and VAChT were highly expressed in the control adrenal medulla, decorating the space between lobules and intermingled between individual chromaffin cells within lobules. The staining intensity was significantly attenuated in Cx36 −/− mice ( n =21 glands from 11 animals, P <0.05 versus WT, n =22 glands from 11 mice, unpaired Student’s t -test), suggesting an impairment of cholinergic presynaptic terminal function. To further address whether deficits also occurred postsynaptically, expression of mRNA encoding nAChR subunits was evaluated by real-time RT-PCR. None of the five tested subunits (α3, α7, α9, β2 and β4) was differentially expressed in Cx36 −/− mice when compared with wild-type mice ( Fig. 9b ). 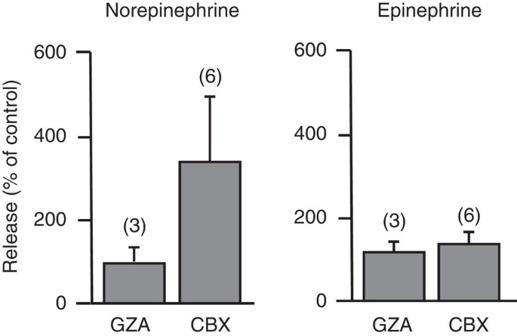Figure 8: Impaired catecholamine secretion in Cx36−/−mice. High frequency splanchnic nerve stimulation does not evoke a significant increase in catecholamine secretion neither in CBX- nor in GZA-treated mice (Mann–WhitneyU-test,n=3 GZA- and 6 CBX-injected mice. Values represent mean±s.e.m.). Figure 8: Impaired catecholamine secretion in Cx36 −/− mice. High frequency splanchnic nerve stimulation does not evoke a significant increase in catecholamine secretion neither in CBX- nor in GZA-treated mice (Mann–Whitney U- test, n =3 GZA- and 6 CBX-injected mice. Values represent mean±s.e.m.). 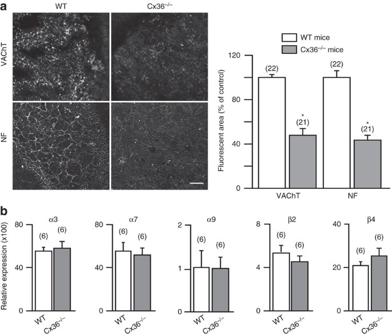Figure 9: Deficits occurring at the splanchnic nerve-chromaffin cell synapse in Cx36−/−mice. (a) Robust decrease of both vesicular acetylcholine transporter (VAChT) and neurofilament (NF) immunostaining in Cx36−/−compared with WT mice. Scale bar, 100 μm. *P<0.05 versus WT, unpaired Student’st-test,n=22 glands from 11 WT mice and 21 glands from 11 Cx36−/−mice. Values represent mean±s.e.m. (b) No change in the expression level of transcripts encoding five nicotinic acetylcholine receptor subunits in Cx36−/−mice (n=6) compared with WT mice (n=6, Mann–WhitneyU-test). Values represent mean±s.e.m. Full size image Figure 9: Deficits occurring at the splanchnic nerve-chromaffin cell synapse in Cx36 −/− mice. ( a ) Robust decrease of both vesicular acetylcholine transporter (VAChT) and neurofilament (NF) immunostaining in Cx36 −/− compared with WT mice. Scale bar, 100 μm. * P <0.05 versus WT, unpaired Student’s t- test, n =22 glands from 11 WT mice and 21 glands from 11 Cx36 −/− mice. Values represent mean±s.e.m. ( b ) No change in the expression level of transcripts encoding five nicotinic acetylcholine receptor subunits in Cx36 −/− mice ( n =6) compared with WT mice ( n =6, Mann–Whitney U- test). Values represent mean±s.e.m. Full size image Our study reports in vivo basal and splanchnic nerve stimulation-evoked catecholamine secretion from the adrenal gland in an anaesthetised mouse. In addition, using a combination of in vivo monitoring of adrenal catecholamine secretion and splanchnic nerve stimulation, we shed light on the functional relevance of gap junctions in the adrenal medullary tissue. It becomes now unquestionable that gap junctions contribute positively to nerve-evoked catecholamine release. A striking observation is that the spontaneous electrical activity in the adrenal medullary tissue in vivo was sporadic and bursting, contrasting with the high frequency firing observed ex vivo [13] , [19] or in cultured chromaffin cells [20] , [21] , [22] . Although our in vivo conditions were designed to minimally disrupt adrenal function, we cannot rule out the possibility that the firing pattern recorded in an anaesthetised animal is attenuated. The bursting pattern is likely to be physiologically relevant as catecholamine release from the adrenal is known to be optimized when nerve impulses are delivered in bursts rather than continuously [23] , [24] . More importantly, we observed that electrical activity was suppressed when action potential propagation along the splanchnic nerve was prevented by TTX. This indicates a predominant nerve-driven activity and a sparse spontaneous electrical firing of chromaffin cells. This finding strengthens the conclusion that chromaffin cell firing discharge is prevailingly paced by synaptic inputs. However, it contrasts with observations made in vitro [25] , [26] , [27] and ex vivo [13] , [19] , in which adrenal chromaffin cells were disconnected from their sympathetic inputs and exhibited a sustained autorhythmic activity [20] supporting robust spontaneous action potential firing. The TTX sensitivity of in vivo spontaneous activity is in agreement with Petrovic et al. [28] , who demonstrated that spontaneous catecholamine release in an adrenal medulla slice is markedly decreased by hexamethonium, indicating that release does not result from spontaneous chromaffin cells activity but rather from the commonly observed spontaneous activation of synaptic inputs [4] , [5] , [12] . The electrical chromaffin cell response to nerve-evoked stimulation was also robustly reduced by hexamethonium, supporting a dominant contribution of nAChRs over muscarinic receptors. This corroborates previous findings in mouse acute slices reporting an inhibition of catecholamine release by hexamethonium [28] , [29] . However, it contrasts with a study performed in hemisectioned mouse adrenal, in which catecholamine release evoked by acetylcholine mainly depended on muscarinic receptors [19] . In previous in vivo measurements of basal and stimulated adrenal catecholamine release, E and NE were alternatively assayed from adrenal-venous blood or from the general blood circulation. In addition, the specie, collection technique and stimulation protocols varied from one study to the other, thus precluding trivial quantitative comparison. Basal and splanchnic nerve stimulation-evoked release of adrenal catecholamines has been directly measured in adrenal-venous blood only in a few cases, in the cat [30] , [31] , rat [15] , [23] , [32] , [33] and dog [34] , [35] but not in the mouse. Our in vivo data indicate a basal E:NE ratio close to 10:1 in the mouse. This is consistent with previously reported ratios ranging from 2 to 7 (refs 15 , 31 , 33 , 34 , 35 ). It is noteworthy that it is the opposite when catecholamines are assayed in the plasma, in anaesthetised animals [30] , [33] , [35] , [36] , including mouse [37] , [38] , [39] , [40] . In response to electrical splanchnic nerve stimulation (0.1 and 4 Hz), adrenal catecholamine output significantly increased with stimulation frequency. In particular, HF stimulation vigorously enhanced the release of both E and NE, as reported in other species [15] , [23] , [24] , [30] , [34] . E and NE can be differentially released from the adrenal, depending on splanchnic nerve stimulation frequency. Whereas NE is the main hormone secreted during LF stimulation (1–5 Hz) in cat [31] , [41] , our results in mouse are in favour of a preferential E secretion at both LF and HF stimulation. The same is observed in rat [15] and dog [35] . The stimulation frequency-dependent increase in catecholamines is a robust event, since it also occurs in acute adrenal slices [42] . In cold-stressed mice, basal catecholamine concentration in adrenal-venous blood was unexpectedly lower than that in control mice. This mismatches with previous data reporting a rise in catecholamine concentration in the adrenal vein in response to various stressors [33] , [36] , [43] . This also contrasts with the typical in vivo increase in catecholamine concentrations measured in plasma, in response to stressful situations [33] , [36] , [40] , [44] . However, the situation in the adrenal-venous blood appears more intricate, such that a robust catecholamine increase detected in plasma is not always associated with equally vigorous catecholamine amounts flowed from the adrenal [44] . The low basal catecholamine concentration we found here was unlikely due to depletion of adrenal catecholamine resources, since the gland further secreted in response to nerve stimulation. Alternatively, the anaesthesia and surgical procedure may have uncontrolled consequences on the basal release. Although ketamine does not modify basal catecholamine secretion [45] , a direct measurement of plasma catecholamines, in a freely moving mouse submitted or not to various stress paradigms, will be necessary to definitely answer this question. Although a direct cell–cell communication through gap junctions has been described in many endocrine/neuroendocrine tissues [46] , [47] , [48] , [49] , including the adrenal medulla [6] , [7] , [11] , its contribution to hormone secretion in vivo has been unambiguously established so far only for insulin [50] , [51] and renin [49] , [52] . Very recent studies performed in the anterior pituitary [53] , [54] strongly support a crucial role for gap junctions in endocrine tissue output, suggesting that the plasticity of gap junction-coupled endocrine cell network is a key element underlying functional adaptation of hormone release at the population level. More remarkable is the observation that functional adaptation to specific hormonal demand persists within the coupled network [55] . If transposed to the chromaffin cell network, this could be particularly relevant in terms of functional tissue adaptation in response to repeated stressful conditions. Regarding the adrenal gland, contribution of gap junctions to stimulation-secretion coupling was previously inferred from in situ experiments in rodent adrenal acute slices [11] , [56] . Conversely, Petrovic et al. [28] reported that gap junctions do not contribute to catecholamine release evoked by localized electrical stimulation. However, the mechanisms engaged when a bipolar electrode is positioned on top of a slice are probably hardly comparable to those involved in the response to distant stimulation of the splanchnic nerve and propagation of action potentials along sympathetic axons. Our in vivo observation that CBX or MFQ decreases nerve stimulation-evoked catecholamine release in conditions in which they prevent intercellular diffusion of fluorescent dyes within the adrenal gland is a strong indication for a role of gap junctions in catecholamine release. Furthermore, this finding is reinforced by demonstration of a more robust effect of CBX on catecholamine secretion in cold-stressed mice, in which the medullary gap junctional communication is upregulated. Unfortunately, in the reverse experiment in which Cx36-built gap junctions were reduced by genetic manipulation, nerve-evoked release was reduced so much that the contribution of gap junctions could not be reliably evaluated. It is noticeable that gap junctions contribute chiefly to NE release in control animals and to both E and NE release in stressed animals. The observation that CBX decreased the release evoked by high frequency stimulation, but not low frequency stimulation, suggests a dominant contribution of connexin-dependent signalling in emergency conditions when the hormonal demand is high. As previously reported [6] , our data identified Cx36 as the ascendant connexin expressed in the mouse medullary tissue and documented the expression of Cx29 transcript. At least two findings support a role of gap junctional communication in catecholamine secretion in mouse. First, we show here that Cx36 and Cx29 are upregulated after an episode of cold stress, as reported for Cx36 and Cx43 in rat [14] . Second, PACAP, a splanchnic-derived peptide transmitter that is released during elevated nerve firing [10] , enhances gap junction-mediated electrical coupling in the mouse adrenal medulla [57] . The most surprising result concerns the considerable decrease of nerve stimulation-evoked catecholamine release in the adrenal medulla of Cx36 −/− mice. The underlying default likely occurs presynaptically, as suggested by the substantial reduction of both NF and VAChT immunolabelling. Although connexin-dependent signalling and chemical synaptic neurotransmission interact with each other in various neuronal tissues [58] , including in the adrenal medulla [6] , [7] , [59] , our finding reveals an unanticipated role for Cx36 at the splanchnic nerve-chromaffin cell synapse. During postnatal development, downregulation of adrenal gap junctional communication parallels the acquisition of the neurogenic control of catecholamine secretion [4] , [12] . In adults, gap junctional communication is under a tonic inhibitory control by cholinergic neurotransmission [5] , [12] . In view of this mutual regulation, one would have expected the lack of gap junctions in Cx36 −/− mice to help implementation of cholinergic nerve fibres rather than to prevent it. The impairment of nerve stimulation-evoked catecholamine release and the decreased expression of NF and VAChT are strong and correlative indications of a degraded innervation of chromaffin cells in Cx36 −/− mice. Defective propagation of signals generated by sympathetic nerve stimulation has been also observed in Cx32-deficient mice [60] . More recently, alterations in physiological properties of neurons via early postnatal blockade of gap junctional communication have been reported, thus shoring up the idea that Cx36 deletion may cause changes in presynapses [61] . This opens intriguing questions as to the inter-relationship between gap junctions and synapses, especially during the early phases of neuronal development. Altogether, the present study ultimately demonstrates that gap junctions are indeed positively contributing to adrenal excitation-secretion coupling in vivo . The contribution of connexin-dependent signalling seems particularly decisive when the organism demand in catecholamines increases. Our study substantiates previous data showing that, in the adrenal medulla, synaptic transmission and gap junctional communication act in synergy to ensure a secretory response appropriate to the organism need. In addition to being the first report demonstrating a regulation of gap junction-mediated cell-to-cell communication in the adrenal medullary tissue in vivo , our study sheds light on the contributions of gap junctions to neurosecretory function. Importantly, our findings might be extended to other neuroendocrine tissues. Indeed, its ubiquitous distribution merits that gap junction-mediated coupling be revisited in most neurosecretory tissues as our study suggests that it is a defining characteristic of endocrine/neuroendocrine organ function in vivo . Animal preparation and surgery All procedures conformed to the animal welfare guidelines of the European Community and were approved by the French Ministry of Agriculture (authorizations No. 34.128 and 49.247). Experiments were performed on 2-month-old male C57BL/6J and Cx36-deficient mice [62] , acclimatised (12 h light-dark cycle, 22 °C) for a minimum of 7 days before use. For in vivo experiments, mice were anaesthetised with ketamine (100 mg kg −1 ) and xylazine (10 mg kg −1 ), i.p. in 160 μl NaCl (9‰). The surgery started with a laparotomy; visceral organs were gently shifted on the right side of the animal to uncover the left adrenal gland. The renal vein and the conjunctive tissue containing the splanchnic nerve were isolated. The splanchnic nerve was placed on a home-made bipolar stimulation electrode. The renal vein was ligated on both the kidney and vena cava sides and then cannulated with a heparinised (20 U ml −1 ) catheter to form a reservoir collecting the blood flowing from the left adrenal ( Supplementary Fig. S1 and Supplementary Movie 1 ). Blood collection and catecholamine assay Twenty minutes after surgery, two blood samples were successively collected during 2 or 5 min each, depending on the stimulation protocol, one control first (C) and then a test one (T) during stimulation. Stimulation-evoked catecholamine release was expressed as the T/C ratio. Samples were centrifugated at 4 °C (7,000 g , 10 min) and stored at −20 °C until use. Catecholamines (epinephrine and norepinephrine) were assayed from 7 μl of plasma using a 2-CAT ELISA KIT (Mediane Diagnostics, Plaisir, France) [63] . Arterial blood pressure measurement Systolic blood pressure (SBP) was measured by tail-cuff plethysmography (BP-2000 blood pressure analysis system, Visitech Systems, Bioseb, Chaville, France) in ketamine/xylazine anaesthetised mice. Mice were introduced into a restraint device with the blood pressure measure cuff placed on the base of the tail. The thermal heating pad underneath was set to 30 °C. SBP and cardiac frequency were monitored every minute for 60 min (15 min as a control period before injection and up to 40–45 min after injection as the test period), to reliably compare the results with adrenal-venous blood catecholamine levels assayed 40–50 min after drug injection). Electrophysiology Square electrical pulses (10 V, 160 ms) were applied to the nerve at low (0.1 Hz, 5 min) or high frequency (4 Hz, 2 min). To block nerve conduction, a tetrodotoxin (TTX)-soaked cotton bud (3 μM) was applied on the nerve, as far as possible (2–3 mm) from the gland. Extracellular recordings were performed with a glass microelectrode (in mM: 150 NaCl, 12.5 KCl, 10 HEPES, pH 7.4). The recording site was located by injection of Chicago Sky Blue 6B (2%, Supplementary Fig. S2 ). In some experiments, the recording electrode contained hexamethonium (200 μM) to impair cholinergic neurotransmission. In vivo blockade of gap junctions Mice were injected i.p. (120 μl NaCl 9‰) before the surgical procedure with either carbenoxolone [64] (CBX, 100 mg kg −1 ) or its inactive analogue glycyrrhizic acid [65] (GZA, 135 mg kg −1 ). In some experiments, mice were injected with the Cx36 uncoupling agent mefloquine [17] (MFQ, 25 mg kg −1 in 75 μl DMSO+H 2 O, 75/25 v/v) or with the vehicle (DMSO+H 2 O, 75/25 v/v). Scrape-loading dye transfer In vivo surgery and pharmacological treatments were identical to those described above. Excised glands were included in agarose, cooled on ice, hemisectioned and incubated for 45 s either in Lucifer yellow (LY, lithium salt; 0.2% in NaCl 9‰, charge -2/MW 457) or Cadaverine (Alexa Fluor 594-conjugated, 50 μM in NaCl 9‰, charge +1/MW 807) [66] . Hemi-glands were immediately fixed in PFA (4% in 0.1 M phosphate buffer) and stored at 4 °C. Hemi-glands were sliced (50 μm) and imaged with an epifluorescence microscope and the ImageJ software. Average light intensity was measured in the adrenal medulla, along an axis perpendicular to the cutting edge (distance=0 at the edge and increasing with penetration into the medulla), leading to a ‘fluorescence versus distance’ curve. Results were further expressed as the area under the curve for statistical analysis. Connexin immunolabelling To process for connexin immunostaining, adrenal glands were rapidly removed from an anaesthetised mouse, embedded in Tissue-Tek O.C.T compound and frozen by immersion in isopentane. The glands were next cut into 20 μm-thick sections using a cryostat. Gland sections were mounted on coverslips, post-fixed at −20 °C for 10 min in acetone and incubated overnight with a rabbit anti-Cx36 or a rabbit anti-Cx43 (1:250; Zymed Laboratories, CliniSciences, Montrouge, France, Cat N°364600 and 483000) polyclonal antibody. Sections were then rinsed and incubated for 2 h at room temperature with a rabbit secondary antibody conjugated to Cy3 (1:2,000; Jackson ImmunoResearch Laboratories, West Grove, PA, Cat N°711-166-152). Primary and secondary antibodies were diluted in PBS containing 2% BSA and 0.1% Triton X-100. Negative controls were performed by omitting primary antibodies. Stained sections were imaged with an epifluorescence microscope (Axoimager, Zeiss, × 20 objective). The fluorescence was quantified with Volocity software (Perkin Elmer, Courtaboeuf, France), the total surface of fluorescent areas positive for connexins (number of fluorescent pixels) was divided by the surface (total number of pixels) of the gland, and expressed as a percentage. Vesicular ACh transporter and neurofilament immunolabelling Adrenal glands were rapidly removed from anaesthetised mice, immediately fixed in PFA (4% in 0.1 M phosphate buffer, 2 h, room temperature) and then stored at 4 °C until processing. Glands were then sliced (50 μm thickness) using a vibratome. Slices were first incubated in mouse FAB IgG (1:200, Eurobio-AbCys, Les Ulis, France, Cat N°BI 3013C) for 2 h at room temperature and then in a rabbit anti-VACht (1:500, Synaptic systems, Goettingen, Germany, Cat N°130 103) polyclonal antibody and a mouse anti-neurofilament 200 (clone N52, 1:500, Sigma, Cat N°NO142) monoclonal antibody for 48 h at 4 °C. Slices were then rinsed and incubated for 2 h at room temperature with a rabbit secondary antibody conjugated to Cy3 and a mouse secondary antibody conjugated to Cy5 (both at 1:2,000; Jackson ImmunoResearch Laboratories, West Grove, PA, Cat N° 711-166-152 and 711-496-152). Primary and secondary antibodies were diluted in PBS containing 2% BSA and 0.1% Triton X-100. Negative controls were performed by omitting primary antibodies. Images acquisition was performed using a LSM 510 Meta confocal microscope (Zeiss, Le Pecq, France) and quantification with the image J software. Quantification of mRNA expression by real-time RT-PCR Total RNA was extracted from macrodissected mouse adrenal medulla using the RNeasy Micro extraction kit (Qiagen, Courtaboeuf, France). RNA (200 ng) was first reverse transcribed using the QuantiTect Reverse Transcription kit (Qiagen) in a final volume of 10 μl. Real-time PCR analyses of the target genes Gjc3 , Gjd2 , Gja1, Chrna3 , Chrna7 , Chrna9, Chrnb2, Chrnb4 and the reference genes Gusb , Hprt and Gapdh were performed using Sybr Green PCR master mix (Applied Biosystems, Foster City, CA) with 1:60 of the reverse-transcription reaction, and were carried out on an ABI 7500 SDS Real-Time PCR system (Applied Biosystems). Primer sequences are given in Supplementary Table S1 , and the concentration used was 300 nM for all genes. After an initial denaturation step for 10 min at 95 °C, the thermal cycling conditions were 40 cycles at 95 °C for 15 s and 60 °C for 1 min. Each sample value was determined from duplicate measurements. Expression of the target transcripts was normalized to the mean of the expression level of the three reference genes according to the formula E=2 −(Ct[Target]−Ctmean[Reference]) , where Ct is the threshold cycle. Solutions and chemicals Xylazine and ketamine chlorhydrate were from Alcyon (Pau, France), Alexa Fluor 594-Cadaverine from Life Technologies (Saint Aubin, France) and mefloquine hydrochloride from BioBlocks, (San Diego, CA). All other compounds were purchased from Sigma. Statistics Numerical data are expressed as the mean±s.e.m. Differences between groups were assessed using the non-parametric Mann–Whitney-test. The effects of nerve stimulation frequency on catecholamine release was assessed using two-way analysis of variance (followed by Bonferroni’s post hoc test). Unpaired Student’s t -test was used to compare means. Differences with P <0.05 were considered significant. How to cite this article: Desarménien, M. G. et al. Gap junction signalling is a stress-regulated component of adrenal neuroendocrine stimulus-secretion coupling in vivo . Nat. Commun. 4:2938 doi: 10.1038/ncomms3938 (2013).